Low MITF/AXL ratio predicts early resistance to multiple targeted drugs in melanoma Increased expression of the Microphthalmia-associated transcription factor (MITF) contributes to melanoma progression and resistance to BRAF pathway inhibition. Here we show that the lack of MITF is associated with more severe resistance to a range of inhibitors, while its presence is required for robust drug responses. Both in primary and acquired resistance, MITF levels inversely correlate with the expression of several activated receptor tyrosine kinases, most frequently AXL. The MITF-low/AXL-high/drug-resistance phenotype is common among mutant BRAF and NRAS melanoma cell lines. The dichotomous behaviour of MITF in drug response is corroborated in vemurafenib-resistant biopsies, including MITF-high and -low clones in a relapsed patient. Furthermore, drug cocktails containing AXL inhibitor enhance melanoma cell elimination by BRAF or ERK inhibition. Our results demonstrate that a low MITF/AXL ratio predicts early resistance to multiple targeted drugs, and warrant clinical validation of AXL inhibitors to combat resistance of BRAF and NRAS mutant MITF-low melanomas. The discovery of the activating BRAF V600E mutation in roughly half of the melanomas [1] has spurred the development of targeted therapies, which are associated with unprecedented clinical benefits. The small-molecule inhibitor vemurafenib, specifically targeting the mutant BRAF V600E kinase, was the first standard of care for patients diagnosed with mutant BRAF metastatic melanoma [2] , [3] , [4] . Although this compound initially reduces tumour burden dramatically, eventually melanomas become resistant and tumours progress while on treatment [5] . Resistance to this treatment occurs by acquisition of additional mutations or other alterations that affect the mitogen-activated protein kinase (MAPK) pathway by either direct [6] , [7] , [8] or indirect signalling [6] , [9] , [10] , [11] . Many resistance mechanisms somehow lead to reactivation of extracellular signal-regulated kinase (ERK), thereby restoring signalling of the oncogenic BRAF/MEK/ERK pathway [12] . In addition, PI3K pathway activation contributes to resistance to BRAF inhibition [13] . Less frequent but equally important to the phenomenon of targeted drug resistance is the observation that ~15–20% of BRAF mutant melanoma patients fail to respond to BRAF inhibition already early on treatment, owing to intrinsic resistance. These patients have little therapeutic options, unless immunotherapy can be given [14] , [15] . On the basis of the frequent occurrence of MAPK pathway reactivation, causing resistance to BRAF inhibition, the clinical rationale arose for combined treatment of BRAF and MEK inhibitors. In a phase 1/2 clinical trial, the median progression-free survival by the BRAF inhibitor dabrafenib and the MEK inhibitor trametinib was extended from 5.8 months on dabrafenib monotherapy to 9.4 months [16] . However, also resistance to the combinatorial therapy eventually develops, leading to rapid disease recurrence. Recently, an ERK inhibitor (SCH772984) with a dual mechanism of action was developed. It inhibits the enzymatic activity of ERK as well as its phosphorylation, and hence activation, by MEK [17] . SCH772984 effectively blocks the proliferation of BRAF and BRAF/MEK inhibitor-resistant cells and has therefore been proposed as a new line of treatment for BRAF mutant (resistant) melanoma. Despite its promise, we considered it conceivable that melanomas will eventually also overcome the cytotoxicity mediated by ERK inhibition. Therefore, we performed a gain-of-function insertional mutagenesis screen to identify possible resistance mechanisms towards ERK inhibition. We identified an insertion in the MITF (Microphthalmia-associated transcription factor) locus, causing sharp upregulation of the corresponding master lineage transcription factor. MITF is responsible for pigmentation and indispensable for the development of the melanocytic lineage [18] . Its expression is usually maintained in melanoma, although MITF-negative specimens exist [19] . The role of MITF in melanoma development and progression is equivocal. For example, high levels of MITF have been reported to block proliferation by the upregulation of cell cycle inhibitors [20] , [21] . In seeming contrast, MITF was found to be amplified in 15% of metastatic melanomas, conceivably reflecting its oncogenic role [22] . Moreover, cells negative for MITF are known to display invasive properties [19] . In an attempt to reconcile these findings, a rheostat model has been proposed [19] . This pieces together three different phenotypes of melanoma cells that are dependent on MITF expression, ranging from differentiation (high MITF), proliferation (moderate MITF) and invasion (low MITF). Our finding that increased MITF expression causes resistance to ERK inhibition is consistent with a recent report showing that MITF is sufficient to render melanoma cells resistant to MEK or ERK inhibitor-induced cell death [9] , [23] . However, those results do not speak to several seemingly opposite functions that have also been attributed to MITF. Therefore, we report here a more in-depth study in melanoma cell lines and clinical specimens to investigate the contribution of MITF expression to the response of melanomas to clinically relevant inhibitors. Overexpressed MITF protects cells against ERK inhibition To identify proteins conferring resistance to MAPK pathway inhibition, we used the recently available ERK inhibitor SCH772984 (ref. 17 ) in a lentiviral Validation-Based Insertional Mutagenesis (VBIM) screen system [24] . Carrying a green fluorescent protein-sequence and a strong CMV promoter, this virus integrates randomly into the genome, resulting in the activation of downstream sequences. This vector comes in three variants to integrate in the three possible open reading frames. Successful integrations lead to the overexpression of FLAG-tagged proteins and can be excised by 4-hydroxytamoxifen (4-OHT)-induced activation of Cre. We used a low-passage human BRAF V600E mutant melanoma cell line (04.07), which is intermediately sensitive to SCH772984 (not all cells are killed by the ERK inhibitor even when used at a high concentration; Supplementary Fig. 1A ). We infected this cell line with the three versions of the insertional mutagenesis vector (SD1–3; Supplementary Fig. 1B ). After 3 weeks of culturing in the presence of 1 μM SCH772984, we were able to pick drug-resistant clones, which were individually expanded. We first confirmed that the resistance occurred owing to an insertion, providing a selective and reversible advantage in the presence of ERK inhibition, as resistance could be reverted by 4-OHT-treatment ( Supplementary Fig. 1C ). In the majority of the clones, we detected one or more Flag-tagged proteins, indicating that successful in-frame insertions had occurred into the genome, leading to overexpression of fusion proteins ( Fig. 1a ). 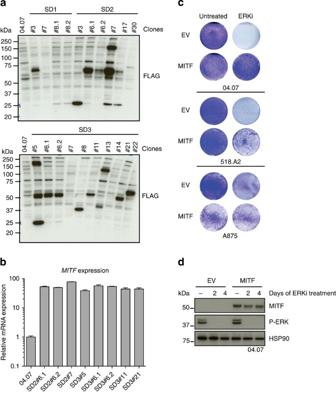Figure 1: Overexpressed MITF protects cells against ERK inhibition. (a) An insertional mutagenesis screen was performed using the VBIM system. A BRAF mutant melanoma cell line of low passage (04.07) was infected with three VBIM vectors (SD1–3; to cover the three reading frames) and treated with 1 μM of the ERK inhibitor SCH772984. Drug-resistant clones were established and analysed for FLAG-tagged proteins resulting from the integration of the viral cassettes. (b) Integration of the VBIM cassettes resulted in MITF overexpression in six independent ERKi-resistant clones, as shown by qRT–PCR, compared with parental 04.07 cells. Note that only clones derived from separate plates were considered as independent clones. Error bars denote s.d. for technical replicates. (c) Lentiviral overexpression of MITF resulted in increased resistance to long-term ERK inhibition in three independent BRAF mutant melanoma cell lines as shown by crystal violet staining. (d) Immunoblot of 04.07 cells confirmed MITF overexpression and inactivation of ERK after inhibitor treatment. HSP90 served as a loading control. Figure 1: Overexpressed MITF protects cells against ERK inhibition. ( a ) An insertional mutagenesis screen was performed using the VBIM system. A BRAF mutant melanoma cell line of low passage (04.07) was infected with three VBIM vectors (SD1–3; to cover the three reading frames) and treated with 1 μM of the ERK inhibitor SCH772984. Drug-resistant clones were established and analysed for FLAG-tagged proteins resulting from the integration of the viral cassettes. ( b ) Integration of the VBIM cassettes resulted in MITF overexpression in six independent ERKi-resistant clones, as shown by qRT–PCR, compared with parental 04.07 cells. Note that only clones derived from separate plates were considered as independent clones. Error bars denote s.d. for technical replicates. ( c ) Lentiviral overexpression of MITF resulted in increased resistance to long-term ERK inhibition in three independent BRAF mutant melanoma cell lines as shown by crystal violet staining. ( d ) Immunoblot of 04.07 cells confirmed MITF overexpression and inactivation of ERK after inhibitor treatment. HSP90 served as a loading control. Full size image We observed an ~55 kDa FLAG-tagged protein in multiple independent clones, raising the possibility that a common gene was activated. Using splinkerette PCR followed by Sanger sequencing, we identified an insertion in intron 2–3 of the MITF gene locus ( Supplementary Fig. 1D ). This finding was confirmed by qPCR, showing up to 100-fold overexpression of MITF , and immunoblotting of six individual clones ( Fig. 1b and Supplementary Fig. 1E ). To functionally validate if MITF can induce resistance to ERK inhibition, we overexpressed it in a panel of melanoma cell lines using a lentiviral system. Exogenous overexpression of MITF promoted the survival and proliferation in three independent BRAF V600E melanoma cells lines in the presence of ERK inhibitor ( Fig. 1c ), despite complete ERK-pathway inhibition ( Fig. 1d ). The same protective effect of MITF was seen for the preclinical BRAF inhibitor PLX4720 or a MEK inhibitor (trametinib or GSK1120212; Supplementary Fig. 1F ). These observations are in agreement with, and extend, recent findings on the role of MITF in the response to MEK and ERK inhibitors [9] , [23] . MITF loss occurs in acquired resistance in vitro and in vivo To determine the regulation of MITF expression during acquired resistance, we generated several cell lines that are resistant to 1 μM SCH772984 ( Supplementary Fig. 2A ) or 3 μM PLX4720 ( Fig. 2a and Supplementary Fig. 2B ) by culturing under increasing drug exposure. In line with our findings from the VBIM screen, we observed either the maintenance of high MITF expression or a moderate increase in MITF expression in three out of seven PLX4720-resistant lines (888mel, A375, D10; Fig. 2b ), along with increased expression of several MITF targets and more pigmentation of the cells. 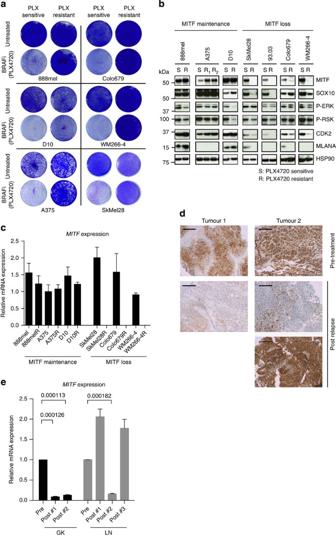Figure 2: MITF loss occurs in acquired resistancein vitroandin vivo. (a) Treatment-naïve BRAF mutant melanoma cells were under constant treatment with PLX4720 until resistance was achieved. Crystal violet staining confirmed resistance to 3 μM PLX4720 in resistant cells in comparison with their sensitive counterparts. (b) Immunoblot of sensitive (S) and resistant (R) melanoma cells showed expression of MITF and MITF-regulated proteins. HSP90 served as a loading control. (c)MITFmRNA expression was measured by qRT–PCR in treatment-naïve and resistant melanoma cell lines normalized toRPL13mRNA expression. Error bars denote s.d. for technical replicates. (d) Human melanoma biopsies (obtained from patients before vemurafenib treatment (pre) and after relapse had occurred (post)) were stained for MITF. Tumour 2 was from a patient with distinct relapsed tumour clones. Scale bars, 200 μm. (e)MITF-MmRNA was measured in human biopsies before vemurafenib treatment (pre) and after relapse had occurred (post) from two different patients. Values were normalized toGAPDHmRNA expression.Pvalues, by paired Student’st-test across triplicates, were only shown for samples for whichMITFmRNA expression dropped. Error bars denote s.d. for technical triplicates. Figure 2: MITF loss occurs in acquired resistance in vitro and in vivo. ( a ) Treatment-naïve BRAF mutant melanoma cells were under constant treatment with PLX4720 until resistance was achieved. Crystal violet staining confirmed resistance to 3 μM PLX4720 in resistant cells in comparison with their sensitive counterparts. ( b ) Immunoblot of sensitive (S) and resistant (R) melanoma cells showed expression of MITF and MITF-regulated proteins. HSP90 served as a loading control. ( c ) MITF mRNA expression was measured by qRT–PCR in treatment-naïve and resistant melanoma cell lines normalized to RPL13 mRNA expression. Error bars denote s.d. for technical replicates. ( d ) Human melanoma biopsies (obtained from patients before vemurafenib treatment (pre) and after relapse had occurred (post)) were stained for MITF. Tumour 2 was from a patient with distinct relapsed tumour clones. Scale bars, 200 μm. ( e ) MITF-M mRNA was measured in human biopsies before vemurafenib treatment (pre) and after relapse had occurred (post) from two different patients. Values were normalized to GAPDH mRNA expression. P values, by paired Student’s t -test across triplicates, were only shown for samples for which MITF mRNA expression dropped. Error bars denote s.d. for technical triplicates. Full size image In contrast, four out of seven PLX4720-resistant lines (SkMel28, Colo679, WM266-4 and 93.03) had downregulated MITF expression to almost undetectable levels relative to their parental counterparts ( Fig. 2b ). In almost all resistant cell lines, ERK and RSK were reactivated to the levels seen in their untreated counterparts. Similarly, four out of six cell lines resistant to 1 μM SCH772984 had decreased expression of MITF accompanied by decreased expression of several target genes ( Supplementary Fig. 2A ). The loss of MITF occurred at the transcriptional level; in fact, the MITF mRNA levels were undetectable, as measured by quantitative reverse transcription-PCR (qRT–PCR) analysis ( Fig. 2c ). Thus, one set of acquired drug-resistant cell lines maintained or increased MITF expression; we call these MITF acq_maint cells. In contrast, for at least half of the cell lines we observed the opposite: a sharp downregulation of MITF expression; we call these MITF acq_loss cells. The differential regulation of MITF during the acquisition of drug resistance suggests that there are two classes of MITF-expressing melanoma cell lines, which differ in their response to MAPK pathway inhibition: in MITF acq_maint cells, MITF signalling is maintained or even induced, potentially contributing to drug resistance. In MITF acq_loss cells, in which MITF is downregulated, maintenance of MITF expression is not required for drug resistance. To study the dynamics of MITF downregulation in relation to the acquisition of a resistant phenotype, two independent MITF acq_loss melanoma cell lines from an independent panel (M229 and M238; ref. 13 ) were permanently exposed to 1 μM vemurafenib and monitored over time. MITF expression sharply dropped on short-term exposure to PLX4720 and was further decreased in the remaining drug-tolerant population, drug-tolerant proliferating population and in resistant cells ( Supplementary Fig. 2C,D ). These results show that acquired resistance is accompanied by a rapid decrease in MITF, and confirm that this is regulated at the transcriptional level. To corroborate these in vitro findings in a physiologically more relevant setting, we performed immunohistochemical staining for MITF on a limited set of human melanoma biopsies. The samples were taken from patients before treatment with vemurafenib and after patients had relapsed with vemurafenib-resistant tumours. In one out of four matched (pre-treatment and post-relapse) sample sets, we observed a sharp drop in MITF abundance ( Fig. 2d , tumour 1). For another patient, we observed a remarkable differential response: while there was abundant expression in the pre-treatment sample, one relapsed melanoma metastasis showed elevated levels of MITF, whereas another had lost detectable expression in most of the resistant tumour cells ( Fig. 2d , tumour 2). These results are in agreement with our in vitro findings and indicate that melanoma drug resistance in vivo is associated not only with gain of MITF expression but also with its loss, even in different relapsed tumour clones from the same patient. To validate these observations in an independent set of BRAF V600E mutant melanomas, we compared MITF mRNA levels before treatment and after resistance had occurred. Again, we found that MITF expression strongly decreased in several resistant tumour clones compared with their treatment-naïve counterparts ( Fig. 2e ). In this cohort of 12 patients who developed resistance to vemurafenib treatment, three relapsed with one or more tumours that significantly decreased in MITF expression (25%). The entire cohort comprised 29 vemurafenib-resistant relapses, of which four displayed a significant downregulation of MITF at the mRNA level. In comparison, in five patients, tumours with elevated MITF expression were found. Thus, MITF acq_maint and MITF acq_loss cells co-exist in vivo and the loss of MITF is commonly seen in the context of MAPK pathway inhibition, both in vitro and in vivo . MITF loss causes cross-resistance to MAPK pathway inhibition To further characterize the differences between the MITF acq_maint and MITF acq_loss cells, we exposed them to several inhibitors of the MAPK pathway, either alone or in combination. PLX4720-resistant MITF acq_maint cells were resistant to another BRAF inhibitor (dabrafenib) but were as responsive to MEK or ERK inhibition as their drug-sensitive counterparts ( Fig. 3a , top). In contrast, PLX4720-resistant MITF acq_loss cells displayed cross-resistance to the full panel of MAPK pathway inhibitors, even when BRAF and MEK were inhibited simultaneously ( Fig. 3a , bottom). Phosphorylation of ERK was similarly suppressed across all cell lines, demonstrating that in all cases the drugs were equally effective towards their respective targets ( Fig. 3b ). In contrast, only PLX4720-resistant MITF acq_maint cells underwent apoptosis on drug treatment as demonstrated by PARP cleavage, whereas MITF acq_loss cells did not display any sign of apoptosis. In a larger set of melanoma cell lines, comparing three MITF acq_maint and three MITF acq_loss cell lines, we observed that the latter group tolerated exposure to higher drug concentrations than MITF acq_maint cells, and hence are more prone to develop cross-resistance ( Fig. 3c , Supplementary Fig. 2G,H ). 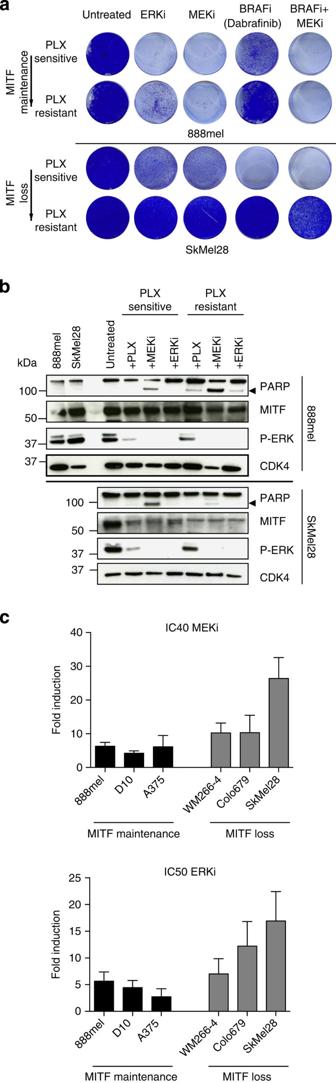Figure 3: MITF loss causes cross-resistance to MAPK pathway inhibition. (a) Two PLX4720-resistant cell lines (888mel and SkMel28) and their treatment-naïve counterparts were treated with either the ERKi SCH772984 (0.5 μM), the MEKi trametinib (0.3 μM), BRAF inhibitor dabrafenib (3 μM) or a combination as indicated and stained with crystal violet after 6 days of treatment. (b) Immunoblotting for the indicated proteins confirmed the downregulation of the MAPK pathway (as judged by P-ERK) and showed cleaved PARP (arrow) as a measure of apoptosis of the cell lines used ina. CDK4 served as a loading control. (c) Six PLX4720-resistant cell lines and their treatment-naïve counterparts were separated in groups that either lose or maintain (or increase) MITF expression on acquiring resistance. These cells were exposed to the MEKi trametinib or the ERKi SCH772984 in dose–response curves. IC40 (for MEKi) or IC50 (for ERKi) were calculated from the curves. Fold increase in IC40 or IC50 was determined comparing resistant to sensitive cells. Mean was calculated from three independent experiments, error bars indicate s.d. Figure 3: MITF loss causes cross-resistance to MAPK pathway inhibition. ( a ) Two PLX4720-resistant cell lines (888mel and SkMel28) and their treatment-naïve counterparts were treated with either the ERKi SCH772984 (0.5 μM), the MEKi trametinib (0.3 μM), BRAF inhibitor dabrafenib (3 μM) or a combination as indicated and stained with crystal violet after 6 days of treatment. ( b ) Immunoblotting for the indicated proteins confirmed the downregulation of the MAPK pathway (as judged by P-ERK) and showed cleaved PARP (arrow) as a measure of apoptosis of the cell lines used in a . CDK4 served as a loading control. ( c ) Six PLX4720-resistant cell lines and their treatment-naïve counterparts were separated in groups that either lose or maintain (or increase) MITF expression on acquiring resistance. These cells were exposed to the MEKi trametinib or the ERKi SCH772984 in dose–response curves. IC40 (for MEKi) or IC50 (for ERKi) were calculated from the curves. Fold increase in IC40 or IC50 was determined comparing resistant to sensitive cells. Mean was calculated from three independent experiments, error bars indicate s.d. Full size image Loss of MITF is accompanied by increased invasiveness In melanoma, low MITF expression has been associated with a phenotypic switch, including increased invasiveness [19] . To determine whether MITF acq_loss cells show such properties, we transferred them to a matrigel-coated chamber and monitored their invasive potential. Indeed, MITF acq_loss cells were endowed with increased invasive capacity when compared to MITF acq_maint cells ( Fig. 4a,b ). In MITF acq_loss cell lines that expressed E-Cadherin before drug exposure, this epithelial protein was lost on the acquisition of drug resistance ( Fig. 4c ). In WM266-4 cells in which E-Cadherin protein expression was below detection level, a decrease in CDH1 mRNA was detected by qRT–PCR ( Supplementary Fig. 2F ). N-Cadherin was more abundant in MITF acq_loss cells already before treatment but remained unaltered after resistance occurred ( Fig. 4c and Supplementary Fig. 2F ). We further investigated additional epithelial to mesenchymal transition (EMT) markers, including the transcription factors ZEB1 and ZEB2 , and found a remarkable downregulation in ZEB2 expression in three MITF acq_loss cell lines and a concomitant increase of ZEB1 in two of the three cell lines ( Fig. 4d ). In WM266-4 cells, instead, TWIST mRNA was highly elevated in resistant cells compared with treatment-naïve ones, suggesting that it might compensate for ZEB1 in mediating EMT and invasion ( Supplementary Fig. 2E ). Further, Dia1 has been described to be downregulated in MITF-dependent invasion [19] . DIA1 mRNA transcription had dropped in two of three MITF acq_loss cell lines ( Fig. 4e ). In addition, the transcription factor Fra-1, which we recently demonstrated to be involved in invasion and metastasis [25] , was increased in all three MITF acq_loss cells ( Fig. 4c ). To determine if the resistance-induced invasiveness was mediated by Fra-1, we introduced Fra-1 knockdown vectors into two MITF acq_loss cell lines ( Fig. 4f ). The depletion of Fra-1 expression decreased the invasive capacity of these cells without affecting cell proliferation ( Fig. 4g,h ). Thus, in addition to displaying a MAPK pathway inhibition cross-resistant phenotype, MITF acq_loss cells are much more invasive than MITF acq_maint cells, which occurs in a Fra-1-dependent manner, and they display properties of EMT. 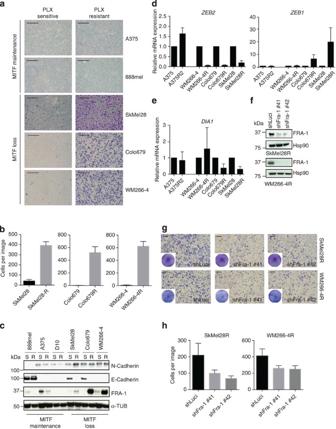Figure 4: Loss of MITF is accompanied by increased invasiveness. (a) PLX4720-resistant melanoma cells and their treatment-naïve counterparts were seeded on a matrigel-coated invasion chamber for 12 h. Cells that invaded through the matrix were stained with crystal violet. Scale bars, 500 μm. (b) Quantification ofafrom at least five images. (c) PLX4720-resistant cells (R) and their treatment-naïve (S) counterparts were blotted for EMT markers.α-Tubulin served as a loading control. (d)ZEB1andZEB2mRNA were measured in acquired PLX4720-resistant cells and their treatment-naïve counterparts. The results are based on three independent experiments and normalized toRPL13. Data are shown as mean+s.d. (e) mRNA expression ofDia1was measured in acquired PLX4720-resistant cells and their treatment-naïve counterparts. The results are based on three independent experiments and normalized toRPL13. Data are shown as mean +s.d. (f) Knockdown of Fra-1 in two PLX4720-resistant cell lines was documented on immunoblot. HSP90 served as a loading control. (g) Two PLX4720-resistant melanoma cells transduced with Fra-1 knockdown and control cells were seeded on a matrigel-coated invasion chamber for 12 h. Cells that invaded through the matrix were stained with crystal violet. Inserts show proliferation in 12 h on polystyrene culture dishes. Scale bars, 200 μm. (h) Quantification ofgof at least five images. Figure 4: Loss of MITF is accompanied by increased invasiveness. ( a ) PLX4720-resistant melanoma cells and their treatment-naïve counterparts were seeded on a matrigel-coated invasion chamber for 12 h. Cells that invaded through the matrix were stained with crystal violet. Scale bars, 500 μm. ( b ) Quantification of a from at least five images. ( c ) PLX4720-resistant cells (R) and their treatment-naïve (S) counterparts were blotted for EMT markers. α -Tubulin served as a loading control. ( d ) ZEB1 and ZEB2 mRNA were measured in acquired PLX4720-resistant cells and their treatment-naïve counterparts. The results are based on three independent experiments and normalized to RPL13 . Data are shown as mean+s.d. ( e ) mRNA expression of Dia1 was measured in acquired PLX4720-resistant cells and their treatment-naïve counterparts. The results are based on three independent experiments and normalized to RPL13 . Data are shown as mean +s.d. ( f ) Knockdown of Fra-1 in two PLX4720-resistant cell lines was documented on immunoblot. HSP90 served as a loading control. ( g ) Two PLX4720-resistant melanoma cells transduced with Fra-1 knockdown and control cells were seeded on a matrigel-coated invasion chamber for 12 h. Cells that invaded through the matrix were stained with crystal violet. Inserts show proliferation in 12 h on polystyrene culture dishes. Scale bars, 200 μm. ( h ) Quantification of g of at least five images. Full size image Absence of MITF marks intrinsically insensitive cells The above experiments focused on the regulation and role of MITF in the context of acquired targeted drug resistance. Next we investigated the impact of different levels of endogenous MITF expression on treatment-naïve melanoma cells regarding sensitivity to MAPK pathway inhibition. For that, we grouped BRAF mutant melanoma cells in ‘MITF endo_hi ’ and ‘MITF endo_lo ’ cells based on their endogenous protein expression levels ( Fig. 5a ) and transcript expression ( Supplementary Fig. 3A ). As expected, most MITF endo_hi cell lines expressed MITF-target gene products like CDK2 and MelanA, whereas those proteins were expressed to lower or even undetectable levels in MITF endo_lo cells. 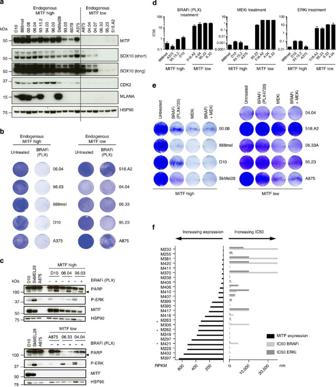Figure 5: Absence of MITF marks intrinsically insensitive cells. (a) Treatment-naïve BRAF mutant melanoma cells were grouped based on their MITF expression by immunoblotting, also for additional proteins as indicated. HSP90 served as a loading control. (b) BRAF mutant melanoma cells were plated at low density and treated with 5 μM PLX4720 for 6 days or left untreated and stained with crystal violet. (c) For a subset of the cells lines fromb, MAPK pathway inhibition and apoptosis indicated by cleaved PARP (arrow) after 3 days of treatment with 5 μM PLX4720 was confirmed by immunoblotting. HSP90 served as a loading control. (d) Sensitivity of MITFendo_hiand MITFendo_lotreatment-naïve melanoma cell lines to the BRAFi PLX4720, to the ERKi SCH772984 and to the MEKi trametinib was determined in dose–response curves. Mean was calculated from three independent experiments, error bars indicate s.d. (e) MITFendo_hiand MITFendo_loBRAFV600Emutant melanoma cell lines were plated at low density and treated with either BRAFi (2 μM), MEKi trametinib (0.1 μM) or a combination. After 6 days, cells were stained with crystal violet. (f) An independent set of treatment-naïve BRAFV600Emutant melanoma cell lines was grouped based on MITF expression, and resistance to the BRAFi (vemurafenib) and the ERKi SCH772984 was determined by dose–response curves. Cell lines withMITFamplification are marked with an asterix. Figure 5: Absence of MITF marks intrinsically insensitive cells. ( a ) Treatment-naïve BRAF mutant melanoma cells were grouped based on their MITF expression by immunoblotting, also for additional proteins as indicated. HSP90 served as a loading control. ( b ) BRAF mutant melanoma cells were plated at low density and treated with 5 μM PLX4720 for 6 days or left untreated and stained with crystal violet. ( c ) For a subset of the cells lines from b , MAPK pathway inhibition and apoptosis indicated by cleaved PARP (arrow) after 3 days of treatment with 5 μM PLX4720 was confirmed by immunoblotting. HSP90 served as a loading control. ( d ) Sensitivity of MITF endo_hi and MITF endo_lo treatment-naïve melanoma cell lines to the BRAFi PLX4720, to the ERKi SCH772984 and to the MEKi trametinib was determined in dose–response curves. Mean was calculated from three independent experiments, error bars indicate s.d. ( e ) MITF endo_hi and MITF endo_lo BRAF V600E mutant melanoma cell lines were plated at low density and treated with either BRAFi (2 μM), MEKi trametinib (0.1 μM) or a combination. After 6 days, cells were stained with crystal violet. ( f ) An independent set of treatment-naïve BRAF V600E mutant melanoma cell lines was grouped based on MITF expression, and resistance to the BRAFi (vemurafenib) and the ERKi SCH772984 was determined by dose–response curves. Cell lines with MITF amplification are marked with an asterix. Full size image We then determined the spectrum of drug sensitivity among a panel of MITF endo_lo and MITF endo_hi cells. On exposure to 5 μM PLX4720 for 6 days, there was a clear survival benefit of MITF endo_lo cells, as illustrated by viability assays and PARP cleavage ( Fig. 5b,c ) This difference was not caused by insufficient pathway inhibition since ERK phosphorylation was diminished irrespective of MITF status. In agreement, comparing four MITF endo_hi with four MITF endo_lo cell lines, the latter showed a dramatic increase in resistance to MEKi as was illustrated by an up to 1,000-fold increase in IC50 values ( Fig. 5d and Supplementary Fig. 3B ). This phenomenon was also seen on combinational inhibition of BRAF and MEK, indicating a much more robust drug resistance phenotype of MITF endo_lo cells than MITF endo_hi cells ( Fig. 5e ). Seeking whether these findings could be confirmed in an independent data set, we investigated MITF expression and drug sensitivity in an additional panel of human BRAF V600E mutant melanoma cell lines. Again we observed an inverse correlation between endogenous MITF expression and the IC50 values for vemurafenib and ERK inhibitor treatment ( Fig. 5f ). AXL and other RTKs are inversely correlated with MITF To identify proteins that are responsible for protecting MITF endo_lo cells from MAPK pathway inhibition, we performed next-generation RNA sequencing on three MITF endo_lo and three MITF endo_hi BRAF V600E cell lines. We found that several receptor tyrosine kinases (RTKs) were expressed to higher levels in the MITF endo_lo cell lines, including AXL, epidermal growth factor receptor (EGFR) and platelet-derived growth factor receptor (PDGFRβ; Fig. 6a and Supplementary Fig. 4A ). Encouraged by these findings, we compared the phosphorylation status of RTKs in an MITF endo_lo and an MITF endo_hi cell line. Already in the untreated control, a subset of RTKs was activated in MITF endo_lo cells ( Fig. 6b , upper array). Exposure for 2 days to 5 μM PLX4720 further increased the activation of several RTKs in MITF endo_lo cells, whereas only a minor activation of RTKs could be detected in MITF endo_hi cells ( Fig. 6b , lower array). In addition to activation, we observed increased expression levels of particularly AXL, PDGFRβ and EGFR in MITF endo_lo cells compared with MITF endo_hi cells in a larger set of melanoma cell lines ( Fig. 6c ). In an independent data set (from Fig. 5f ), we correlated MITF and AXL mRNA expression and observed a significant inverse correlation (correlation coefficient of −0.84 and correlation P -value of 7E −09 ; Supplementary Fig. 4B ). In addition, this data set validated the increased resistance to BRAF and ERK inhibition in MITF-low/AXL-high cells. To confirm these findings in vivo , we extracted protein from patient-derived xenografts (PDX)-derived tumour samples and blotted for MITF, MITF targets and RTKs. Similar to our in vitro findings, AXL and PDGFRβ were only expressed in tumours where MITF was absent or expressed at very low levels ( Fig. 6d ). Consistent with these data, analysis of 356 TCGA melanoma transcriptomes supported the anticorrelation between MITF and RTKs including AXL ( Fig. 6e ). 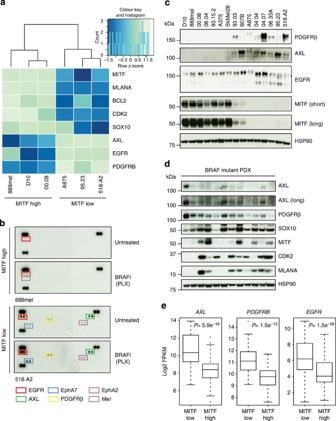Figure 6: AXL and other RTKs are inversely correlated with MITF. (a) RNA sequencing was performed in three MITFendo_hiand three MITFendo_loBRAFV600Emutant melanoma cell lines. The genes in the heatmap were selected based on theMITFexpression, expression of MITF-target genes and expression of the RTKs AXL, EGFR and PDGFRβ. (b) A phospho-RTK array was performed comparing one MITFendo_hiand one MITFendo_lomelanoma cell line untreated or treated with 5 μM PLX4720 for 2 days. (c) MITFendo_hiand MITFendo_locell lines were immunoblotted for the RTKs PDGFRβ, AXL and EGFR. HSP90 served as a loading control. (d) Protein extracts from treatment-naïve BRAF mutant PDX tumours were immunoblotted for the indicated antibodies. (e) Analysis of 356 TCGA melanoma transcriptomes confirming anticorrelation between MITF and RTKs including AXL.Pvalues were computed by a one-sided Wilcoxon ranksum test on the expression levels ofAXL,EGFRandPDGFRBbetween the top quartile (MITF high,n=89) and bottom quartile (MITF low,n=89) ofMITFexpression across the samples. Figure 6: AXL and other RTKs are inversely correlated with MITF. ( a ) RNA sequencing was performed in three MITF endo_hi and three MITF endo_lo BRAF V600E mutant melanoma cell lines. The genes in the heatmap were selected based on the MITF expression, expression of MITF-target genes and expression of the RTKs AXL, EGFR and PDGFRβ. ( b ) A phospho-RTK array was performed comparing one MITF endo_hi and one MITF endo_lo melanoma cell line untreated or treated with 5 μM PLX4720 for 2 days. ( c ) MITF endo_hi and MITF endo_lo cell lines were immunoblotted for the RTKs PDGFRβ, AXL and EGFR. HSP90 served as a loading control. ( d ) Protein extracts from treatment-naïve BRAF mutant PDX tumours were immunoblotted for the indicated antibodies. ( e ) Analysis of 356 TCGA melanoma transcriptomes confirming anticorrelation between MITF and RTKs including AXL. P values were computed by a one-sided Wilcoxon ranksum test on the expression levels of AXL , EGFR and PDGFRB between the top quartile (MITF high, n =89) and bottom quartile (MITF low, n =89) of MITF expression across the samples. Full size image RTK inhibition increases effect of BRAF inhibition These results raised the possibility that high expression of one or more RTKs contributed to the intrinsically resistant phenotype of MITF endo_lo cells. This prompted us to expose melanoma cells to compounds specifically targeting the RTKs AXL, EGFR and PDGFRβ, either alone or in combination. Single inhibition of either AXL or EGFR led to melanoma cell death only at high drug concentration irrespective of their MITF expression ( Supplementary Fig. 4C ). In contrast, the combined treatment of single RTK inhibition with MAPK pathway inhibitors caused a considerable decrease in viability ( Fig. 7a,b ). In a triple combination, treatment of MITF endo_lo cells with AXL, EGFR and PDGFR inhibitors further sensitized MITF endo_lo cells to BRAF inhibition alone or combined BRAF+MEK inhibition ( Fig. 7a,b , Supplementary Fig. 5A,B ). These results confirm that MITF endo_lo cells are highly intrinsically drug resistant. However, at the same time, these data indicate that several RTKs, including AXL, contribute to drug resistance. 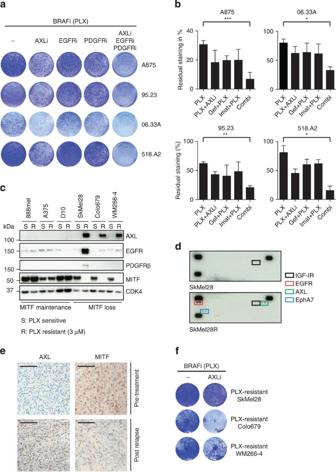Figure 7: RTK inhibition increases effect of BRAF inhibition. (a) MITFendo_locells were exposed to a combination of RTK inhibitors (AXLi R428 (0.3 μM), EGFRi Gefitinib (2 μM) and PDGFRβi Imatinib (1 μM)) and BRAFi PLX4720 (5 μM). After 9 days of combined treatment the remaining cells were stained with crystal violet. (b) Quantification ofa, comprising three independent experiments. Values were normalized to untreated control (100%). Error bars represent s.d.; pairedt-test was performed for statistical analysis, *P<0.05, **P<0.01, ***P<0.001. (c) PLX4720-resistant melanoma cells and their treatment-naïve counterparts were immunoblotted for AXL, EGFR and PDGFRβ. CDK4 served as a loading control. (d) PLX4720-resistant SkMel28 and their naïve counterparts were blotted on a phospho-RTK array. (e) Matched human melanoma biopsies obtained from a patient before vemurafenib treatment (pre) and after relapse had occurred (post) were stained for MITF and AXL. Scale bars, 100 μm. (f) AXL-expressing PLX4720-resistant melanoma cells were exposed to 0.3 μM of the AXL inhibitor R428 for 9 days and the remaining cells stained with crystal violet. Figure 7: RTK inhibition increases effect of BRAF inhibition. ( a ) MITF endo_lo cells were exposed to a combination of RTK inhibitors (AXLi R428 (0.3 μM), EGFRi Gefitinib (2 μM) and PDGFRβi Imatinib (1 μM)) and BRAFi PLX4720 (5 μM). After 9 days of combined treatment the remaining cells were stained with crystal violet. ( b ) Quantification of a , comprising three independent experiments. Values were normalized to untreated control (100%). Error bars represent s.d. ; paired t -test was performed for statistical analysis, * P <0.05, ** P <0.01, *** P <0.001. ( c ) PLX4720-resistant melanoma cells and their treatment-naïve counterparts were immunoblotted for AXL, EGFR and PDGFRβ. CDK4 served as a loading control. ( d ) PLX4720-resistant SkMel28 and their naïve counterparts were blotted on a phospho-RTK array. ( e ) Matched human melanoma biopsies obtained from a patient before vemurafenib treatment (pre) and after relapse had occurred (post) were stained for MITF and AXL. Scale bars, 100 μm. ( f ) AXL-expressing PLX4720-resistant melanoma cells were exposed to 0.3 μM of the AXL inhibitor R428 for 9 days and the remaining cells stained with crystal violet. Full size image Next we determined the expression pattern of these RTKs in the setting of acquired resistance, particularly in PLX4720-sensitive cells and their resistant counterparts. All three MITF acq_loss cell lines examined, which had lost MITF expression after prolonged exposure to PLX4720, showed a strong upregulation of AXL, whereas PDGFRβ and EGFR were upregulated in only one of these cell lines ( Fig. 7c ). Furthermore, MITF acq_loss cells displayed increased phosphorylation of these RTKs, which was not detected before drug resistance was acquired ( Fig. 7d ). Together these results suggest that increased expression and activity of a set of RTKs, particularly AXL, is seen not only in innate but also acquired resistance of melanoma cells. Consistently, in a matched set of pre-treatment and post-relapse samples, the MITF/AXL anticorrelation was recapitulated ( Fig. 7e ). To determine whether AXL inhibition can be used to impact on BRAF V600E mutant melanoma cells resistant to MAPK pathway inhibition, we exposed AXL-expressing PLX4720-resistant cells and their treatment-naïve counterparts to the AXL inhibitor R428. In two of the three resistant cell lines we observed a profound, and in one a modest, decrease in viability on drug treatment ( Fig. 7f ). Taken together, these data indicate that AXL is a key determinant of resistance of melanomas to MAPK pathway inhibition; targeting this RTK in the context of combination therapy is likely to impact on innate or acquired resistant melanomas in the setting of MAPK pathway inhibition. MITF is a predictive biomarker also in NRAS mutant melanomas Finally, to extend our findings to another relevant melanoma subtype, we determined MITF expression in NRAS mutant cells by next-generation RNA sequencing. In a set of eight cell lines, we found MITF to be weakly expressed in four, along with the MITF targets MLANA , BCL2 and CDK2 ( Fig. 8a ). In contrast, the mRNAs encoding AXL, EGFR and PDGFRβ were predominantly expressed in NRAS mutant cells with low MITF expression. These differences in mRNA levels correlated with the expression levels of their corresponding proteins: an inverse correlation between MITF and RTK expression was also observed in NRAS mutant cells, similar to BRAF mutant cells ( Fig. 8b ). Consistently, on a phospho-RTK array, AXL and EGFR showed increased phosphorylation in an NRAS mutant MITF endo_lo cell line ( Fig. 8c ). In addition, we observed an inverse correlation of MITF and AXL mRNA expression in an independent NRAS mutant and BRAF/NRAS wt cell line panel ( Supplementary Fig. 6A ) and in NRAS mutant melanoma PDX ( Supplementary Fig. 6B ). 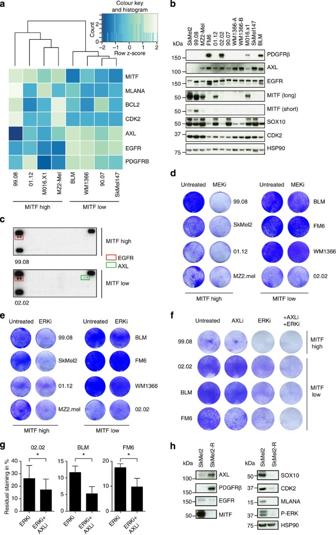Figure 8: MITF is a predictive biomarker also in NRAS mutant melanomas. (a) RNA sequencing was performed on four MITFendo_hiand four MITFendo_loNRAS mutant melanoma cell lines. The genes in the heatmap were selected based on theMITFexpression, expression ofMITF-target genes and expression of the mRNAs coding for the RTKs AXL, EGFR and PDGFRβ. (b) Treatment-naïve NRAS mutant melanoma cells were immunoblotted for MITF, RTKs and other proteins as indicated. HSP90 served as a loading control. WM1366-A/B refers to different batches of the same cell line. (c) A phospho-RTK array was performed comparing one NRAS mutant MITFendo_hiand one MITFendo_lomelanoma cell line. (d,e) MITFendo_hiand MITFendo_loNRAS mutant melanoma cells were plated at low densities and treated with the MEKi trametinib (2.5 nM) (d) or ERKi SCH772984 (0.25 μM) (e) or left untreated for 6 days and stained by crystal violet. (f) Melanoma cells were plated at low density and treated with the AXLi R428 (0.5 μM), the ERKi SCH772984 (1 μM) or in combination. After 6 days of treatment, plates were stained with crystal violet. (g) Quantification off, based on three biological replicates. Error bars represent s.d.; pairedt-test was used for statistical analysis, *P<0.05. (h) A MEKi-resistant NRAS mutant melanoma cell line and its treatment-naïve counterpart were blotted for the indicated proteins. HSP90 served as a loading control. Figure 8: MITF is a predictive biomarker also in NRAS mutant melanomas. ( a ) RNA sequencing was performed on four MITF endo_hi and four MITF endo_lo NRAS mutant melanoma cell lines. The genes in the heatmap were selected based on the MITF expression, expression of MITF -target genes and expression of the mRNAs coding for the RTKs AXL, EGFR and PDGFRβ. ( b ) Treatment-naïve NRAS mutant melanoma cells were immunoblotted for MITF, RTKs and other proteins as indicated. HSP90 served as a loading control. WM1366-A/B refers to different batches of the same cell line. ( c ) A phospho-RTK array was performed comparing one NRAS mutant MITF endo_hi and one MITF endo_lo melanoma cell line. ( d , e ) MITF endo_hi and MITF endo_lo NRAS mutant melanoma cells were plated at low densities and treated with the MEKi trametinib (2.5 nM) ( d ) or ERKi SCH772984 (0.25 μM) ( e ) or left untreated for 6 days and stained by crystal violet. ( f ) Melanoma cells were plated at low density and treated with the AXLi R428 (0.5 μM), the ERKi SCH772984 (1 μM) or in combination. After 6 days of treatment, plates were stained with crystal violet. ( g ) Quantification of f , based on three biological replicates. Error bars represent s.d. ; paired t -test was used for statistical analysis, * P <0.05. ( h ) A MEKi-resistant NRAS mutant melanoma cell line and its treatment-naïve counterpart were blotted for the indicated proteins. HSP90 served as a loading control. Full size image We also examined the sensitivity of these two classes of cell lines to MEK and ERK inhibitors. In full agreement with our observations for BRAF mutant melanoma, NRAS mutant melanoma cells lacking MITF expression were unresponsive to targeted inhibition of MEK ( Fig. 8d ) or ERK ( Fig. 8e ) and resistance correlated with a low MITF/AXL ratio. Combined treatment with ERK and AXL inhibitors of NRAS mutant melanoma cell lines cooperatively decreased viability ( Fig. 8f,g ). To confirm the specificity of R428, we treated NRAS mutant cells with BMS-777607, another inhibitor targeting AXL, and achieved comparable results to R428 ( Supplementary Fig. 6C ). In addition, the knockdown of AXL expression by short hairpins in FM6 cells cooperated with ERK inhibition to kill the drug-resistant population, in a dose-dependent fashion ( Supplementary Fig. 6D ). By continuously increasing the concentration, we made a sensitive MITF endo_high cell line resistant to MEKi ( Supplementary Fig. 6E ); this cell line was cross-resistant to ERKi. We observed a drastic decrease in MITF and MITF-target gene expression, which was accompanied by sharp increases in AXL and PDGFR expression ( Fig. 8h ). Thus, similar to BRAF mutant melanoma cells, NRAS mutant melanoma cells harbouring a low MITF/high AXL ratio are resistant to drugs targeting the MAPK pathway, which can be reversed by co-inhibiting AXL. A large body of evidence has implicated the melanocyte lineage factor MITF not only in melanoma progression but also in drug resistance. For example, MITF is amplified in a subset of human melanomas, ectopically expressed MITF cooperates with mutant BRAF in oncogenic transformation and MITF copy gain correlates with chemoresistance [22] , [26] Furthermore, a germline MITF(E318K) mutation has been suggested to confer increased melanoma susceptibility [27] , [28] , [29] . Consistent with this view, we identified MITF as a locus that was commonly activated in an insertional mutagenesis screen for genes causing resistance to a newly developed ERK inhibitor. Indeed, ectopically expressed MITF caused melanoma cells to become unresponsive to ERK inhibition. In addition, we found MITF levels to be elevated in some PLX4720-resistant cell lines. High-level MITF expression and expression of MITF-target genes have recently been found to play an important role in drug resistance to BRAF inhibition [30] , [31] , to MEK inhibition [23] and combined treatment [9] , [12] . Thus, much of the available evidence points to MITF-driving melanoma progression and contributing to resistance to MAPK pathway inhibition. When pursuing our initial findings on the role of MITF in mediating resistance to ERK inhibition, however, we observed that also the absence of endogenous MITF expression is beneficial for melanoma cells to survive MAPK pathway inhibition, and that, in fact, endogenous MITF expression was required to adequately respond to the inhibitor. Indeed, very low levels or absence of MITF was invariably associated with intrinsic resistance to several inhibitors and cocktails thereof acting across the MAPK pathway in vitro , in BRAF and NRAS mutant melanoma cells alike. Corroborating these results in the context of relapsing melanoma patients, we observed that in a number of human melanomas that had acquired drug resistance, MITF expression was significantly decreased. In one case, we observed a remarkable divergence, with independent relapsing tumour clones displaying either a strong increase, or a sharp decrease, in MITF expression levels relative to the pre-treatment tumour. Our results suggest that either mechanism can account for the acquisition of a drug-resistant phenotype and merit more comprehensive analyses on the role and exact frequency of MITF deregulation in acquired resistance. From a cohort of 12 patients, we found MITF to be downregulated in three patients relapsed with resistant melanoma. In comparison, MITF gain was found in five patients. The total number of tumours that gained MITF expression was higher (eight out of 29 versus four out of 29) although one patient in this cohort alone relapsed with five tumours that gained MITF, and we cannot distinguish if those tumours represented independent events or resulted from a pre-established common resistant clone. Despite a modest frequency of MITF loss based on as-yet limited analysis, we speculate that, due to the increased invasiveness and metastatic potential that MITF-low cells display, MITF downregulation might occur more commonly. This would enable the tumour cells to not only become drug resistant but also to disseminate from the primary tumour. They may regain MITF expression again while forming a secondary tumour, similar to the reversion of EMT downstream in the metastatic cascade, but this needs to be investigated further. Our results suggest that in the context of acquired resistance, at least two distinct classes of melanomas exist: the first maintains or increases MITF expression (denoted here as MITF acq_maint cells); the second class (MITF acq_loss cells), comprising at least half of the cell line panels we studied, sharply downregulates MITF expression on acquiring the resistance trait. Characterizing MITF acq_loss and MITF acq_maint PLX4720-resistant cells, we found that loss of MITF correlated with increased cross-resistance towards MAPK pathway inhibitors. This suggests that MITF loss marks a population of cells that are proliferating and surviving independently of the MAPK pathway. Furthermore, these cells showed increased invasive capacity associated with an EMT-like signature, as marked by a decrease in E-Cadherin. Dia1 mRNA followed the MITF expression pattern in acquired resistance cells, potentially facilitating Rock1-dependent invasiveness [19] . Invasiveness was also associated and partly caused by increased expression of the AP1 family transcription factor Fra-1, which we recently demonstrated to drive a metastatic programme in human breast cancer [25] . These findings are in line with, and extend, a model that has been proposed previously [32] , [33] . It describes a dynamic phenotypic switch between proliferative and invasive states that melanoma cells can undergo to gain invasive properties and metastasize. This idea is consistent with a recent report by Garraway and co-workers [34] , describing a melanoma drug response as a function of transcriptional cell states linked to MITF and NF-κB. Elaborating on this concept, it has been reported that subpopulations of slowly cycling melanoma cells exist, which are marked by the H3K4 demethylase [35] and low MITF levels [36] . The switching phenomenon can be accompanied by loss of MITF and dedifferentiation of primary melanoma cells as marked by loss of MelanA [37] . Furthermore, it has been reported recently that the transcription factors Zeb1 and Zeb2 not only regulate EMT but are expressed in opposed directions in melanocytes, thereby controlling MITF expression and differentiation [38] . Loss of Zeb2 results in dedifferentiation, accompanied by loss of MITF and upregulation of Zeb1, further supporting the idea that acquired resistant cells can lose MITF and dedifferentiate. Our data suggest that therapy-resistant melanoma cells undergo a similar phenotypic switch and dedifferentiation as a function of MITF loss of, marking an invasive subpopulation of resistant cancer cells. In treatment-naïve MITF-low cells, we found a remarkable inverse correlation between the absence of MITF and increased expression levels of several RTKs, predominantly EGFR, PDGFRβ and AXL. Likewise, in acquired resistance, we detected a striking inverse correlation between the loss of MITF and gain of expression of the aforementioned RTKs, particularly AXL. These observations suggest that the expression of these RTKs protects melanoma cells from targeted therapy and that their expression is, either directly or indirectly, negatively regulated by MITF. Recently, SOX10 was identified as a negative regulator of EGFR expression in melanoma, suggesting that loss of SOX10 leads to an increase in EGFR expression leading to acquired resistance [39] . SOX10 can directly transactivate the MITF promoter [40] and cooperates with MITF in activating further downstream targets [41] . However, despite a correlation between SOX10 and MITF expression, we find that absence of MITF and expression of RTKs are not strongly dependent on the absence of SOX10 in treatment-naïve melanoma cells, certainly not in those harbouring NRAS mutation, nor in cells that have acquired resistance. These data suggest that MITF is a central determinant of RTK expression and drug resistance in melanoma. Given the resistance emerging commonly to treatment with single inhibitors of the MAPK pathway, experimental combinatorial therapies have been launched. But early clinical data on BRAF mutant melanoma patients treated with a combinatorial approach of BRAF and MEK inhibitors (dabrafenib+trametinib) indicates that unfortunately, even in that setting eventually most patients become resistant to the treatment [13] , [42] . Thus, addition of an alternative or third compound prolonging clinical response is highly needed. Our results predict that MITF-low melanoma patients, whether harbouring a BRAF or NRAS mutation, may benefit from additional AXL inhibition. We show that single inhibition of AXL strongly decreases viability in two out of three PLX4720-resistant cells even in the absence of the BRAF inhibitor, whereas AXL alone does not affect treatment-naïve cells. In some cases, the pattern is more complex, because in addition to AXL, other RTKs are upregulated. For instance, in PLX4720-resistant SkMel28 cells, we observe in addition to AXL also the upregulation of EGFR and PDGFRβ, likely explaining why AXL inhibition alone was insufficiently cytotoxic for this cell line. These results underscore the strong resistance phenotype of MITF-low melanomas. We propose that the loss of MITF expression marks melanomas that display early resistance to a broad range of targeted inhibitors and cocktails thereof. An inverse correlation between the expressions of MITF and AXL has been reported previously [9] , [43] , [44] . AXL is a tyrosine receptor kinase that is overexpressed in several human cancers including ocular melanoma [45] , [46] , [47] . Interestingly, in addition to its implication in promoting tumour growth, AXL has been reported to induce EMT and metastasis [48] . AXL expression is directly transcriptionally regulated by the Fra-1 transcription factor in bladder cancer [49] . In cells that have acquired resistance, we find coincident increases in Fra-1 and AXL expression and a stronger invasive phenotype, which are accompanied by a decrease in MITF. These results suggest a model for MITF-dependent repression (whether directly or indirectly) of several RTKs. In conclusion, there is a wide body of evidence speaking to MITF driving both melanoma progression and drug resistance, which is consistent with our finding that the overexpression of MITF renders melanomas less susceptible to targeted inhibitors. But we show here that also instead, the loss of MITF marks a melanoma class that is at least as drug resistant, and to a broader range of MAPK pathway and other targeted inhibitors, as cells with amplified MITF. This is associated with high expression (mostly by direct and indirect derepression) and activation of several RTKs. Our results therefore demonstrate that a low MITF/AXL ratio predicts resistance to multiple targeted drugs impacting on the MAPK pathway and RTKs. They also provide a rationale for clinically exploring AXL inhibitors to combat resistance in MITF-low/AXL high, BRAF and NRAS mutant melanomas. Validation-based insertional mutagenesis screen The insertional mutagenesis screen was performed as previously described [24] . In brief, an intermediately sensitive melanoma cell line of low passage (04.07) was infected separately with the three different VBIM constructs (SD1–3) in three 48-well plates (10,000 cells per well). Two days after infection, the cells were transferred to six-well plates. The next day they were exposed to 1 μM SCH772984 for 3 weeks until single colonies had formed. These were picked and cultured individually in the presence of the drug. For identification of insertions, DNA was isolated using DNAzol reagent (Invitrogen). Splinkerette PCR was used according to the published protocol [19] , [24] and subsequently Sanger sequencing was applied on the amplified products. Vectors MITF-M was amplified from human melanocyte cDNA and cloned into pcDHpuro using EcoR1 and Not1 restriction sites. Forward primer: 5′- GGGGAATTCATGGATGCTGGAAATGCTAGAATATAATCACTATCAGG -3′ Reverse primer: 5′- GGGGCGGCCGCCTAACAAGTGTGCTCCGTCTCTTCC -3′ FRA-1 and AXL hairpins were from the TRC library. FRA-1: #41: TRCN0000019541, #42: TRCN0000019542 AXL: #572: TRCN0000000572, #573: TRCN0000000573, #575: TRCN0000000575. qRT–PCR and primers RNA was isolated using Trizol (Ambion), following standard protocol. Reverse transcription was performed with oligo-dT primers. qRT–PCR-primers were designed using Primer3 software. qRT–PCR was performed with SYBR green master mix (Applied Biosystems, Warrington, UK) on a StepOnePlus Real-Time PCR system (Applied Biosystems). RNA levels were normalized against β -ACTIN , GAPDH , TUB4A or RPL13 . The following primers were used: MITF forward: 5′- CAGGCATGAACACACATTCAC -3′ MITF reverse: 5′- TCCATCAAGCCCAAGATTTC -3′ MITF-M forward: 5′- GGAGCTCACAGCGTGTATTTTTCC -3′ MITF-M reverse: 5′- GACTTGGGAATCAAAGTACCTAGTTC -3′ ACTINB forward: 5′- CCAACCGCGAGAAGATGA -3′ ACTINB reverse: 5′- CCAGAGGCGTACAGGATAG -3′ RPL13 forward: 5′- GAGACAGTTCTGCTGAAGAACTGAA -3′ RPL13 reverse: 5′- TCCGGACGGGCATGAC -3′ ZEB1 forward: 5′- TGCACTGAGTGTGGAAAAGC -3′ ZEB1 reverse: 5′- TTGCAGTTTGGGCATTCATA -3′ ZEB2 forward: 5′- AGTACCAGCGGAAACAAGGA -3′ ZEB2 reverse: 5′- TTTTTGCGAGACAGACAGGA -3′ CDH1 forward: 5′- GGCCAGGAAATCACATCCTA -3′ CDH1 reverse: 5′- AGCCAGTTGGCAGTGTCTCT -3′ CDH2 forward: 5′- GGACCGAGAATCACCAAATG -3′ CDH2 reverse: 5′- AGATCTGCAGCGTTCCTGTT -3′ TUBA4A forward: 5′- GACAGCTCTTCCACCCAGAG -3′ TUBA4A reverse: 5′- TGAAGTCCTGTGCACTGGTC -3′ GAPDH forward: 5′- CAATGACCCCTTCATTGACC -3′ GAPDH reverse: 5′- GACAAGCTTCCCGTTCTCAG -3′. Inhibitors and solvents MEK inhibitor GSK1120212/trametinib, BRAF inhibitors PLX4720, PLX4032/vemurafenib and GSK211436/dabrafenib, EGFR inhibitor gefitinib, c-Kit/PDGFR inhibitor imatinib/Gleevec and AXL inhibitor BMS-777607 were all purchased from Selleck Chemicals (Houston, TX, USA). ERK inhibitor SCH772984 was provided by Merck & Co, Whitehouse Station, NJ, USA (under an MTA). AXL inhibitor R428 was from Axon Medchem (Groningen, the Netherlands), the metabolic poison phenyl arsine oxide (PAO) and solvent dimethylsulfoxide were from Sigma-Aldrich (St Louis, MO, USA). All drugs were reconstituted in 100% dimethylsulfoxide to a final concentration of 10–20 mM. Cell lines, cell culture conditions and treatments Melanoma cell lines and HEK293T cells were cultured in DMEM with fetal bovine serum (Sigma), 2 mM glutamine, 100 U ml −1 penicillin and 0.1 mg ml −1 streptomycin (all Gibco) under standard conditions. HEK293T cells were used for virus production for MITF overexpression. In brief, HEK293T cells were transfected with the plasmid of interest and the helper plasmids (pMDLglpRRE, pHCMV-G and pRSVrev). Viral supernatant was either snap frozen or immediately used for infection. Infected melanoma cells were selected with puromycin (Sigma). To generate BRAFi- or ERKi-resistant cells, cells were exposed to increasing concentrations of PLX4720 (up to 3 μM) or SCH772984 (up to 1 μM) and resistance was confirmed by measuring cell viability under treatment. All drug-resistant cell lines were permanently cultured under 3 μM of PLX4720, 1 μM vemurafenib, 1 μM SCH772984 or 0.1 μM GSK211436. For dose–response curves and viability assays, cells were plated and equal concentration of inhibitors was added 1 day after seeding. For short-term viability assays (dose–response curves), cells were plated in a 96-well format and drugs were diluted with the HP D300 Digital Dispenser (Tecan, Giessen, Germany). After 3 to 5 days of incubation, the medium was replaced by a dilution of CellTiter Blue reagent or CellTiter-Glo Luminescent Cell Viability Assay (Promega, Madison, WI) in medium. Two hours later, luminescence was measured by the Infinite M200 microplate reader (Tecan). Long-term viability assays were performed in 6- or 12-well plate format. Inhibitor solutions were replaced every 2 to 3 days and plates were stained with crystal violet after 5 to 9 days of treatment (as indicated). For protein, DNA and RNA analysis, cells were treated on 10-cm dishes and snap frozen after harvesting. Patient-derived xenografts To generate PDX, human melanoma fragments were collected after surgical resection and transplanted subcutaneously into NSG mice. PDX were maintained in mice for subsequent passages. For this, cells from the first passage PDX (X1) were dissociated by 200 U ml −1 collagenase/1 μg ml −1 DNAse incubation for 20 min at 37 °C, filtered through a 70-μm cell strainer, washed, resuspended in matrigel and subcutaneously injected into NSG mice (5 × 10 5 per flank). Alternatively, PDX-derived cell lines (M016) were generated by dissociating tumours and cultured under standard conditions. Invasion assay and Phospho-RTK array To examine the invasive potential 200,000 freshly trypsinized cells were seeded on matrigel-coated chambers (BD Biosciences) in serum-free medium. The lower compartment contained medium supplemented with 9% fetal bovine serum. After overnight incubation, non-invasive cells were removed from the chamber and invaded cells were stained with crystal violet. Pictures of invaded cells were taken on an Axio Vert A1 microscope (Zeiss). Phospho-RTK arrays were performed using the human Phospho-RTK Array from RD Systems (Minneapolis, USA). All steps were performed according to the manufacturer's protocol. Immunohistochemistry EAF-fixed tumour samples were embedded in paraffin and stained with haematoxilin/eosin according to standard procedures. Western blotting and antibodies Cell pellets were lysed in RIPA buffer (50 mM TRIS pH 8.0, 150 mM NaCl, 1% Nonidet P40, 0.5% sodium deoxycholate, 0.1% SDS) supplemented with complete protease inhibitor cocktail (Roche Applied Science) and phosphatase inhibitors 10 mM NaF, 1 mM Na3VO4, 1 mM sodium pyrophosphate, 10 mM beta-glycerophosphate. Protein concentration was determined with the Protein Assay (Bio-Rad). Western blotting was performed with standard techniques using 4–12% Bis-Tris polyacrylamide-SDS gels (NuPAGE, Life Technologies) and nitrocellulose membranes (Whatman, GE Healthcare). Blots were blocked in 4% milk in PBS plus 0.2% Tween 100 and incubated with primary antibodies: Phospho-AKT (1:1,000, sc-7985-R), AXL (1:500, sc-1096), BCL2 (1:1,000, sc-492), CDK2 (1:1,000, sc-163), CDK4 (1:1,000, sc-601), EGFR (1:500, sc-03), FRA-1 (1:1,000, sc-605X) and HSP90 (1:5,000, sc-7947) were purchased from Santa Cruz; E-Cadherin (1:1,000, 610181) and N-Cadherin (1:1,000, 610920) from BD Biosciences; MAP kinase p44/42 Thy202/Tyr204 (1:1,000, 9106), MEK 1/2 phospho (1:1,000, 9154S), PARP (1:1,000, 9542) and PDGFRβ (1:1,000, 3169S) from Cell Signaling; MLANA (1:5,000, MS_716P0) and MITF (1:1,000, MS-771-P1) from Neomarkers; MITF (1:1,000, ab12039) and Sox10 (1:1,000, ab-17732) from Abcam; RSK1 Thr359/Ser363 from Millipore (1:1,000); FLAG (1:1,000, F3165) and α-Tubulin (1:5,000, T9026) from Sigma. The following secondary antibodies were used: swine anti-goat IgG (1:2,000, ALI0404, Biosource), goat anti-rabbit peroxidase conjugate (1:5,000, G21234) and goat anti-mouse (1:5,000, G21040), both purchased from Invitrogen. Western blots were incubated in a 1:1 dilution of solution1 (0.1 M Tris pH 8, 2.5 mM luminol, 0.4 mM p-Coumaric acid, all Sigma) and solution2 (0.1 M Tris pH 8, 30% H 2 O 2 , all Sigma) and chemiluminescent signal was visualized using high performance autoradiography films (Hyperfilm MP, Amersham). RNA-seq analysis Illumina 50 bp paired-end RNA-seq data was collected on a panel of 28 melanoma cell lines. Read mapping was performed using TopHat version 2.0.9 with the NCBI Build 37 reference genome [50] . Read counts per gene were quantified using HTSeq version 0.5.4. Counts were adjusted for gene length and GC content and quantile normalized using the CQN R package to obtain gene level offsets. Read counts were fitted to a generalized linear model with offsets for the final normalization step using the DESeq2 R package [51] . Pearson correlation coefficients between genes for all samples were calculated using R [52] , [53] , [54] . Illumina 90 bp paired-end RNA-seq data was collected on 14 melanoma cell lines. Read mapping was performed using the same approach as for the melanoma cell line panel as described above. Read counts were transformed by applying a variance stabilization with DESeq (1.12.1). In DESeq the dispersion estimate estimateDispersions had parameters: method =‘per-condition’ and fitType =‘local’ and for null model evaluation with no replicates method =‘blind’, and sharingMode =‘fit-only’. Heatmaps were generated with gplots (2.12.1) as available through Bioconductor. Analysis was performed, and plots were made using the statistical programming language R (v 3.0.2). Level 3 RNA sequencing expression values in FPKM for MITF, AXL, EGFR and PDGFRB were downloaded from the TCGA website ( http://cancergenome.nih.gov/ ) for the Skin Cutaneous Melanoma [SKCM] samples. Differential expression was computed by one-sided wilcoxon rank test on the expression distribution of the gene in the MITF-high group (tumour samples in top quartile of MITF expression) and MITF-low group (samples in the bottom quartile of MITF expression). The RNA-seq data are available under accession number GSE61544 and GSE62526. How to cite this article: Müller, J. et al . Low MITF/AXL ratio predicts early resistance to multiple targeted drugs in melanoma. Nat. Commun. 5:5712 doi: 10.1038/ncomms6712 (2014).